Urban characteristics attributable to density-driven tie formation Motivated by empirical evidence on the interplay between geography, population density and societal interaction, we propose a generative process for the evolution of social structure in cities. Our analytical and simulation results predict both super-linear scaling of social-tie density and information contagion as a function of the population. Here we demonstrate that our model provides a robust and accurate fit for the dependency of city characteristics with city-size, ranging from individual-level dyadic interactions (number of acquaintances, volume of communication) to population level variables (contagious disease rates, patenting activity, economic productivity and crime) without the need to appeal to heterogeneity, modularity, specialization or hierarchy. A larger percentage of people live in cities than at any point in human history [1] , while the density of urban areas is generally increasing [2] . One of the enduring paradoxes of urban economics concerns why people continue to move to cities, despite elevated levels of crime, pollution, disease and wage premiums that have steadily lost ground to premiums on rent [3] . New York in the 18th century, according to Thomas Jefferson, was ‘a toilet of all the depravities of human nature’. Since Jefferson’s day, the city has grown to host the depravities of 100-fold more people, yet the stream of new arrivals has not stemmed. While the forces behind any urban migration are complex, the advantages afforded by urban density comprise an important driver. Smith [4] was one of the first to point to urban centres as exceptional aggregators, whether of innovations or depravities. Cities appear to support levels of enterprise impossible in the countryside, and urban areas use resources more efficiently, producing more patents and inventions with fewer roads and services per capita than rural areas [5] , [6] , [7] , [8] , [9] , [10] . Despite the widespread focus on density as a driver for the uniqueness of cities both in scientific and popular audiences, we still lack a compelling generative model for why an agglomeration of people might confer an advantage. Important advances in several fronts have highlighted the difficulty in gaining an understanding of the urban processes beyond the density description level. Early economic models of agglomeration point to the role of technology diffusion in creating intellectual capital [11] , [12] , [13] , but lack a quantitative description of the generative mechanism for how this diffusion happens. Hierarchies have also been proposed as an elegant mechanism for this growth [14] ; however, recent studies hint at the absence of well-defined hierarchy across geographical scales [15] , [16] , [17] , [18] , [19] . It has also been observed [20] that diversity among residents and their intermingling displays a weak correlation with cities' success thus prompting the authors to conclude ‘more fine-scale data on interactions among people of different disciplines—or the culture, laws and peculiarities of cities—is required to better assess the under- or overperformance of innovation of cities’. Recent developments in the study of social networks shed some light on this challenge. Empirical evidence suggests that interactions and information exchange on social networks are often the driving force for idea-creation, productivity and individual prosperity. Examples of this include the theory of weak ties [21] , [22] , structural holes [23] , the strong effect of social interaction on economic and social success [24] , the influence of face-to-face interactions on the effect of productivity, as well as the importance of information flow in the management of Research and Development [25] , [26] . Consequently, it seems that understanding the mechanism of tie formation in cities is the key to the development of a general theory for a city’s growth described by it’s economic indicators and its population. Following this line of thinking, our proposed answer for super-linear growth of cities can be regarded as a natural extension of Krugman's insights on industries [6] . Krugman pointed out the connection between manufacturing efficiency and transportation of goods as a function of proximity of factories. Similarly, our theory connects the efficiency of idea-creation and information flow to the proximity of individuals generating them. These ideas have a long lineage in urban sociology, urban geography and economic geography. Louis Wirth, for example, conceptualized these processes in the late 1930s (ref. 27 ), prompting a vast literature in economic geography that explores the relationship between density and innovation, as well as that between diffusion (via social ties) and population density (going back to Hagerstrand in the 1950s (refs 28 , 29 ); and a more recent, but well-established literature on density and creativity (see, for example, Richard Florida’s work [30] , [31] , [32] ). In this paper, we present a simple, bottom-up, robust model describing the efficient creation of ideas and increased productivity in cities. This contribution’s goal is to integrate these ideas into a single mathematical model that can be tested against available empirical data. Our model consists of two essential features. We propose a simple analytical model for the number of social ties T ( ρ ) formed between individuals, with population density ρ as its single parameter. We demonstrate that increases in density and proximity of populations in cities leads to a super-linear growth of social-tie density for urban population. We then show that the diffusion rate along these ties—a proxy for the amount and speed of information flow and idea adoption—accurately reproduces the empirically measured scaling of urban features such as rate of AIDS/HIV (acquired immunodeficiency syndrome/human immunodeficiency virus) infections, communication and GDP (gross domestic product). The model naturally leads to a super-linear scaling of indicators with city population [9] without the need to resort to any parameter tuning (although it predicts a different functional form than a simple power–law and is a more accurate match to the data). The surprisingly similar scaling exponent across many different urban indicators (see Supplementary Note 1 and Supplementary Table S1 ), suggests a common mechanism behind them. Social-tie density and information flow, therefore, offer a parsimonious, generative link between human communication patterns, human mobility patterns and the characteristics of urban economies, without the need to appeal to hierarchy, specialization or similar social constructs. A model for social-tie density We propose to model the formation of ties between individuals (represented as nodes) at the resolution of urban centres. As our model is based on geography, a natural setting for it is a two-dimensional Euclidean space with nodes denoted by the coordinates on the infinite plane. Furthermore, we also assume that these nodes are distributed uniformly in space, according to a density ρ defined as, ρ =no. of nodes per unit area. While the assumption of uniform density is an approximation, the qualitative features of the model are unaffected by other more realistic choices of the density distribution—see Supplementary Note 2 and Supplementary Fig. S1 . Following Liben-Nowell et al . [33] , we define the probability of a tie to form between two nodes i, j in the plane as where the rank is defined as and d ij is the Euclidean distance between the two nodes. If j lies at a radial distance r from node i, then the number of neighbours closer to i than j is the product of the density and the area of the circle of radius r , and thus the rank is simply, which implies that the probability an individual forms a tie at distance r goes as , similar in spirit to a gravity model [34] . For a randomly chosen node, integrating over r up to an urban mobility ‘boundary’ denoted as r max , we obtain the expected number of social ties for this chosen node denoted as t ( ρ ). where . We note that r max may well be unique for each city, and is often determined by geographical constraints, as well as city infrastructure (cf. Supplementary Note 3 and Supplementary Fig. S2–S3 ). Integrating over the number of social ties for all nodes within a unit area gives us the social-tie density T ( ρ ), with C ′= C −1. Thus the density of social ties formed between individuals grows as , a super-linear scaling consistent with the observations made by Calabrese et al . [35] (also discussed in the content below). We argue that T ( ρ ) to a first approximation is the individual dyadic-level ingredient behind the empirically observed growth of city indicators. For more detail on the theoretical analysis and support for the assumptions involved, see Supplementary Note 4 and 5 and Supplementary Figs S4–S6 . In order to test this theoretical result, we perform simulations of tie formation with more realistic discrete settings. Urban areas differ dramatically in both regional boundaries and population density. It is thus important to test the sensitivity of the model to a diversity of input parameters for the density ρ and the urban ‘boundary’ r max . We start from an empty lattice of size N × N , with N 2 possible locations. The density ρ is gradually increased by randomly assigning new nodes to empty locations on the grid, where each node represents a small community, or city block of 10 2 individuals. Once a node is added, the probability of forming a tie with one of its existing neighbours is computed by counting the number of nodes closer to this node according to equation (1). To test the sensitivity of our results to the relevant parameters we vary the size of the grid (20≤ N ≤400) of blocks to mimic different scales for city boundaries r max assuming r max is the size of the grid. In addition, we also vary city population between 10 4 and 10 7 residents, as well as the functional form of the density distribution. In Fig. 1 we show the average over 30 realizations of the simulation for different values of the grid size N and city boundary r max . The density ρ in this case represents the relative percentage of occupied locations on the grid, and T ( ρ ) the total number of ties formed between nodes. As Fig. 1 shows, the agreement between the theoretical expression for T ( ρ ) equation (5) and the curves generated by the simulation, is excellent at all scales despite our continuum approximation ( R 2 ≈1). 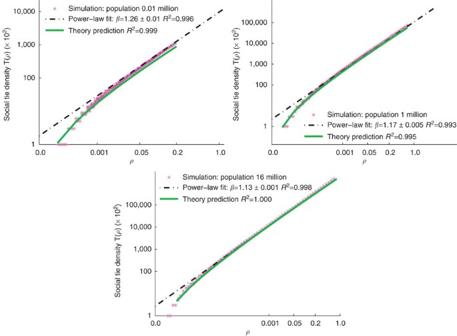Figure 1: The number of social ties as function of grid sizes and urban mobility limits. The number of tiesT(ρ) plotted as a function ofρfor various grid sizesN. The data points represent the average overn=30 realizations of the simulation described in the text, while the solid green line is the theoretical expression equation (5). The dashed line is a fit to the form. As can be seen in each case the agreement between theory and simulation is excellent. The best fit to the scaling exponent yields a value ofβ≈1.15 independent ofN. Note that the measured value of the exponent in empirical data is 1.1≤β≤1.3. Figure 1: The number of social ties as function of grid sizes and urban mobility limits. The number of ties T ( ρ ) plotted as a function of ρ for various grid sizes N . The data points represent the average over n =30 realizations of the simulation described in the text, while the solid green line is the theoretical expression equation (5). The dashed line is a fit to the form . As can be seen in each case the agreement between theory and simulation is excellent. The best fit to the scaling exponent yields a value of β ≈1.15 independent of N . Note that the measured value of the exponent in empirical data is 1.1≤ β ≤1.3. Full size image As a comparative exercise, on the same plot, we also show the best fit to the form and find a value of β ≈1.16. We note that this value is strikingly similar to empirically observed values by fitting a power–law to the relationship between population and urban indicators. It has been suggested that a fit of the form can easily be mistaken for x β (ref. 36 ), which together with our model suggests that the observed scaling of cities may alternatively be described by equation (5). The latter functional form is additionally supported by the fact that it represents a generative model for the emergence of urban features as a result of density-driven communication patterns, without any parameter tuning or a priori assumption about the structure of the underlying social network. Our simulation results indicate that the scaling described in equation (5) is robust with respect to the choice of different functional forms for the density distribution. ( Supplementary Note 2 and Supplementary Fig. 1 ). Empirical evidence for the effect of social-tie density Recent work [35] shows a super-linear relationship between calling volume (time) and population across different counties in the United States. As Fig. 2 illustrates, the super-linear relationship in the data is approximated by the authors as a power–law growth y = ax β with β ≈1.14. However, by assuming a uniform distribution on county sizes and treating population as a proxy for density, we show that our density-driven model is able to capture precisely the distribution of the call volume. The model produces the exact shape of the curve, including the power–law growth pattern ( β =1.14) and tilts on both end, with an adjusted R 2 =0.99 (see Fig. 2 ). Consequently, we propose that the model may well provide a reasonable explanation for communication patterns observed in US counties. 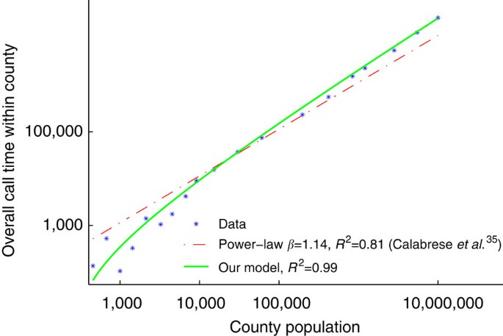Figure 2: Overall time of calls between residents of a county as a function of its population. The points refer to the data (adapted from Calabreseet al.35computed from ten million users’ mobile phone call records within United States during July 2010), while the solid line is the theoretical prediction from the model equation (5) adapted to raw population. The model captures both the super-linear growth and tilts on both ends of the curve while providing a superior fit to the data (based on adjustedR2-value) when compared with a pure power–law relation (dashed curve). Figure 2: Overall time of calls between residents of a county as a function of its population. The points refer to the data (adapted from Calabrese et al . [35] computed from ten million users’ mobile phone call records within United States during July 2010), while the solid line is the theoretical prediction from the model equation (5) adapted to raw population. The model captures both the super-linear growth and tilts on both ends of the curve while providing a superior fit to the data (based on adjusted R 2 -value) when compared with a pure power–law relation (dashed curve). Full size image Information diffusion and adoption with social-tie density We note that the expected patterns of link and interaction formation in itself is insufficient to explain how growth processes in cities work to create observed certain scaling phenomena such as productivity and innovations. Instead, we believe that the manner in which these links spread information and encourage idea and behaviour adoptions actually determines value-creation and productivity. As it is known that social network structure has a dramatic effect on the access of information and ideas [21] , [24] , [23] , [25] , [26] , it seems plausible that higher social-tie density should engender greater levels of idea spreading leading to the observed increases in productivity and innovation. To test the hypothesis that a city’s productivity is related to how far information travels and how fast its citizens gain access to innovations or information, it is natural to examine how this information flow scales with population density, and to quantify the functional relationship between link topology and speed of information spreading. We, therefore, simulated two models of contagion of information diffusion [37] , [38] , [39] on networks generated by our model. The first contagion model simulates diffusion of simple facts, where a single exposure is enough to guarantee transmission. The second more complex diffusion model is typical of behaviour adoption, where multiple exposures to a new influence/idea is required before an individual adopts it. In Fig. 3 , we discover that in both susceptible-infectious (SI) and complex contagion models the mean diffusion speed grows in a super-linear fashion with β ≈1.2, in line with our previous results and match well with the disease spreading indicators in cities [9] . As a consequence we conclude that an explanation for the observed super-linear scaling in productivity with increasing population density is the super-linear scaling of information flow within the social network. 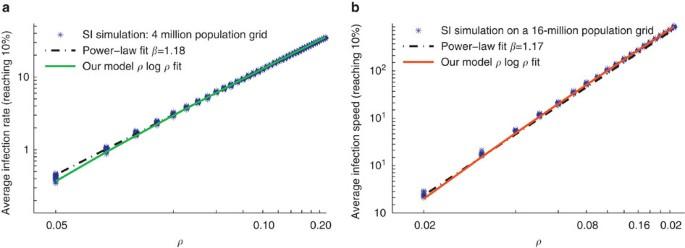Figure 3: The spreading rate as a function of density for two different contagion models. (a) The mean spreading rate as a function of densityρ. The points correspond ton=30 realizations of simulations of the SI model on a 200 × 200 grid. The dashed line corresponds to a fit of the formwithα=0.18. The solid line is a fit to the social-tie density model. (b) The mean spreading rate as a function ofρunder the complex contagion diffusion model based onn=30 realizations of simulations. The dashed line corresponds to the power–law fit of the formwithα=0.17. Once again the solid line is the fit to the model described in the paper. In both cases, the social-tie density model provides a better fit than a simple power–law with with much lower mean-square errors (29% and 41% lower respectively). Figure 3: The spreading rate as a function of density for two different contagion models. ( a ) The mean spreading rate as a function of density ρ . The points correspond to n =30 realizations of simulations of the SI model on a 200 × 200 grid. The dashed line corresponds to a fit of the form with α =0.18. The solid line is a fit to the social-tie density model. ( b ) The mean spreading rate as a function of ρ under the complex contagion diffusion model based on n =30 realizations of simulations. The dashed line corresponds to the power–law fit of the form with α =0.17. Once again the solid line is the fit to the model described in the paper. In both cases, the social-tie density model provides a better fit than a simple power–law with with much lower mean-square errors (29% and 41% lower respectively). Full size image Population level variables While in most cases it is not possible to obtain the social-tie density of a city directly, our model suggests that population density is strongly correlated with social-tie density across cities with similar transportation infrastructure and economic situations (that is, similar r max ). Therefore, we here explore social-tie density indirectly by using population density measures, and we only focus on horizontal comparison of cities of similar levels of economic development, such as US cities and European Union cities. As a test case for our hypothesis, we study the prevalence of AIDS/HIV infections in cities in the United States. In Fig. 4 , we plot the prevalence of AIDS/HIV in 90 metropolitan areas in 2008 (ref. 40 ) as a function of population density. As the figure indicates, there is fairly good agreement between the data and the curve generated by our model of diffusion using both the simple and complex contagion models. 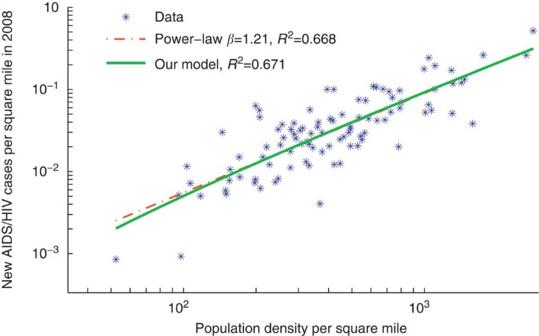Figure 4: Spreading rate of HIV as a function of density in US Metropolitan Statistical Areas. The relationship between density and AIDS/HIV spreading rate of the 90 metropolitan statistical areas from recent Centers for Disease Control and Prevention and US Census surveys. As is visible, the model captures the qualitative trends in the data. Figure 4: Spreading rate of HIV as a function of density in US Metropolitan Statistical Areas. The relationship between density and AIDS/HIV spreading rate of the 90 metropolitan statistical areas from recent Centers for Disease Control and Prevention and US Census surveys. As is visible, the model captures the qualitative trends in the data. Full size image The same agreement holds for European cities on economic indicators. In Fig. 5 , we plot the overall GDP per square km in NUST-2 (Nomenclature of Territorial Units for Statistics level-2) regions in the European Union as a function of population density ρ , as well as population size. The NUST-2 regions are defined by the European Union as the city-size level territorial partition for census and statistics purposes [41] . We find a strong positive correlation between density and the corresponding urban metric with a super-linear scaling component, but conversely a much weak and sublinear growth pattern on raw population size. While it is not the main focus of this paper, we show that the super-linear growth on density can be often be indicated in data as super-linear growth on population, and that density is a better indicator for socio-economic growth than population—see Supplementary Note 4 . 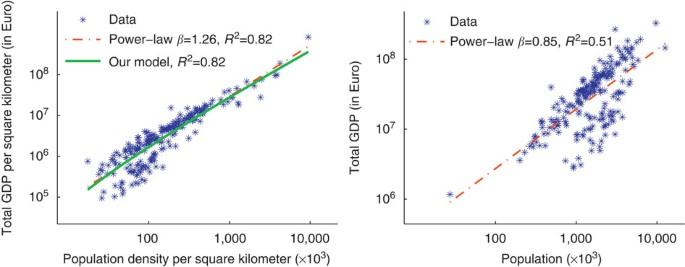Figure 5: Correlation between GDP and population, as well as correlation between GDP and population density for all 247 NUST-2 regions in the European Union. Left panel: correlation between density and GDP, suggesting a strong correlation with a super-linear functional form as predicted by the model. A pure power–law fit to the data is also shown for illustrative purposes. Right panel: the correlation between population and GDP this time showing a sublinear functional form. However, the poorR2-value suggests that raw population does not correlate, as well as density with GDP growth in cities. Figure 5: Correlation between GDP and population, as well as correlation between GDP and population density for all 247 NUST-2 regions in the European Union. Left panel: correlation between density and GDP, suggesting a strong correlation with a super-linear functional form as predicted by the model. A pure power–law fit to the data is also shown for illustrative purposes. Right panel: the correlation between population and GDP this time showing a sublinear functional form. However, the poor R 2 -value suggests that raw population does not correlate, as well as density with GDP growth in cities. Full size image Note that in both data sets the scaling exponents are restricted within a narrow band 1.1≤ β ≤1.3, potentially suggesting a common mechanism behind both the prevalence of AIDS/HIV and scaling of GDP with respect to the population density. An advantage afforded by our model is the need to dispense with parameter tuning, as the model naturally produces this scaling within a reasonable margin of error. Thus, by considering social structure and information/disease flow as a major driving force in many of the city indicators, our approach provides a unique and general theory to the super scaling phenomena of cities. Both the spreading of information (potentially leading to increase productivity and innovation) and contagious diseases rely on the mechanism of social interactions. However, while information can mediate via Mass Media (exogenous) influence, and/or endogenous (word-of-mouth) processes, we chose to highlight the AIDS/HIV spreading data to validate our model, as an example of a purely endogenous process. In this paper, we propose social-tie density (the density of active social ties between city residents) as a key determinant behind the global social structure and flow of information between individuals. Based on this, we have described an empirically grounded generative model of social-tie density to account for the observed scaling behaviour of city indicators as a function of population density. Our model accurately explains how urban density drives the super-linear growth of social interaction density [35] , and eventually the super-linear growth of productivity as observed in many empirical data sets. The conceptual distinction between density and social density is an important one, as it has been missing in popular accounts that may percolate to urban planners and policy-makers. As a matter of fact, throughout the 20th century, the United States has witnessed major shifts from dense to suburban, then back to dense urban planning. As recently as 1970, suburban populations surpassed the urban one—motivated by a search for an idealized small, low-density, locally oriented community [42] . Indeed, these back and forth shifts may have been facilitated by an incomplete understanding of the benefits afforded by urban density. The model predicts that social-tie density scales super-linearly with population density, while naturally accounting for the narrow band of scaling exponents empirically observed across multiple features and different geographies. We note that this is achieved without the need to resort to parameter tuning or assumptions about heterogeneity, modularity, social hierarchies, specialization or similar social constructs. We, therefore, suggest that population density, rather than population size per se, is at the root of the extraordinary nature of urban centres. As a single example, metropolitan Tokyo has roughly the same population as Siberia while showing remarkable variance in criminal profile, energy usage and economic productivity. We provide empirical evidence based on studies of indicators in European and American cities (both categories representing comparable economic development), demonstrating that density is a superior metric than population size in explaining various urban indicators. We note that current technology makes remote communication and collaboration extremely easy and convenient; however, the importance of packing people physically close to each other is still widely emphasized [43] , [44] , [45] . We postulate that cities potentially operate under the same principle–as a consequence of proximity and easy face-to-face access between individuals— communication and ultimately productivity is greatly enhanced. Thus, though it is reasonable to surmise that individuals migrate to the city for reasons connected with individual needs and preferences, our argument suggests that, it is the benefits afforded by social-tie density that maintains them as residents. While our model provides a fundamental first-principles basis for explaining productivity of cities, we note the importance of higher-order variables such as transportation infrastructure in order to tailor the model to specific cases to get better results. As an example, the density of social ties is intrinsically a function of the ease of access between residents living in the same city. Consider the case of Beijing, which has a very high population density, but due to its traffic jams, is currently de-facto divided into many smaller cities with limited transportation capacities between them. Consequently, it may not demonstrate a higher social-tie density than other cities with a much lower population density. Thus a direct comparison of the model predictions with a similarly dense area such as Manhattan needs to take into account this refinement. In keeping with the spirit of the simplicity and bottom-up approach of our model, we chose to use data from cities within the United States and the European Union such that extraneous variables are controlled for. A number of theories of urban growth suggest the importance of specialist service industries, or high-value-add workers, as generative models of city development. While our model does not disprove these theories, it provides a plausible and empirically grounded model that does not require the presence of these special social structures. The other theories must, therefore, appeal to different sorts of data in order to support their claims. Cities are one of most exceptional and enduring of human inventions. Most great cities are exceptions in their own right: a New Yorker feels out of place in Los Angeles, Paris or Shanghai. However, this exceptionalism may be more due to our attention to human-scale details than to the underlying structures. In this paper, we have presented a generative theory that accounts for observed scaling in urban growth as a function of social-tie density and the diffusion of information across those ties. It is our hope that this provides both a foundation for the commonalities across all cities and a beginning point for which divergence between specific cities can be explored. Data sets All data sets used for analysis in this paper are publicly available. We collected data from the official websites of US Centre for Disease Control and Prevention, US Census Bureau and the Statistical Office of the European Union. The detailed information for each data set is provided in the paper. Diffusion models Assuming that the spread of information and disease are archetypes of simple contagions, for the simple exposure contagion case, we run the SI model [37] , [38] on networks generated by our model, and measure the speed at which the infection reaches a finite fraction of the population. We start by generating networks according to the process described in the introduction and then randomly pick 1% of the nodes as seeds (that is, initial infected nodes). The probability of an infection at a given time-step, to spread from an infected to a susceptible node, is denoted as ε , which we fix to be ε =1 × 10 −2 . The simulation terminates at the point when 10% of the population is in the infected state. The networks generated are snapshots at different densities ρ and as before we vary the size of the grid N . For the complex contagion case, we adopt the complex contagion model [39] . We assume that 10% of the population follows a simple contagion process: an individual can be infected by a single infected neighbour; the remaining 90% of the population follows a complex contagion process: an individual is infected, if at least two of its neighbours are infected. The rest of the simulation is identical to the simulation with the SI model, and we measure the time steps required to infect 10% of the population. Denoting S ( ρ ) as the number of time steps taken to infect 10% of the population, the mean spreading rate R ( ρ ) shown in Fig. 3 is computed using: Assuming that the mean spreading rate is proportional to the network density (that is, R ( ρ ) T ( ρ )), we also fit the data to the form where k is a constant and T ( ρ ) follows from equation (5). (Cf. Supplementary Note 6 and Supplementary Fig. S7 ). How to cite this article: Pan, W. et al . Urban characteristics attributable to density-driven tie formation. Nat. Commun. 4:1961 doi: 10.1038/ncomms2961 (2013).